Cooperation between different RNA virus genomes produces a new phenotype An RNA virus population generally evolves rapidly under selection pressure, because of high error rates of the viral RNA polymerase. Measles virus, an enveloped RNA virus, has a fusion protein mediating fusion of the viral envelope with the cell membrane. Here we observe that a non-fusogenic recombinant measles virus evolves, after passages, into mutant viruses which regain the ability to induce membrane fusion. Unexpectedly, we identify a mutant virus possessing two types of genomes within a single virion: one genome encoding the wild-type fusion protein, the other a mutant version with a single amino-acid substitution. Neither the wild-type nor mutant protein by itself is able to mediate membrane fusion, but both together exhibit enhanced fusion activity through hetero-oligomer formation. Our results reveal a molecular mechanism for the ‘cooperation’ between different RNA virus genomes, which may have implications in viral evolution and in the evolution of other macromolecules. An RNA virus population generally evolves rapidly under selection pressure, because of the high error rate of viral RNA polymerase [1] , [2] , [3] , [4] , [5] . This feature of RNA viruses is thought to have an important role in viral pathogenesis and survival under selection pressure, exemplified in the evolution of the human immunodeficiency virus and the hepatitis C virus [3] , [5] , [6] , [7] . The high mutation rate may allow these viruses to develop resistance to host immune responses and antiviral drugs, a major complication in the efforts to control their infection. Measles is an acute contagious viral disease characterized by high fever and a maculopapular rash, and remains a major cause of infant death in developing countries [8] . In rare cases, persistent infection in the central nervous system causes lethal subacute sclerosing panencephalitis, several years after acute infection. Measles virus (MV), the causative agent, is an enveloped RNA virus in the family Paramyxoviridae . MV has two envelope glycoproteins, a receptor-binding hemagglutinin (H) and a fusion (F) protein mediating fusion of the viral envelope with the cell membrane. Binding of the MV H protein to a cellular receptor is thought to trigger conformational changes in the neighbouring F protein, leading to virion-to-cell fusion or cell-to-cell fusion (syncytium formation) in infected cells [9] . During our study on the mechanism of MV entry, we accidentally found ‘cooperation’, a new form of viral evolution dependent on a mixture of two different RNA virus genomes, and revealed the molecular mechanism for this phenomenon. Fusion assay inconsistent with one recombinant virus To facilitate our studies on MV entry, we produced the enhanced green fluorescent protein (EGFP)-expressing recombinant MV that has the H protein fused with the FLAG-TEV-MYC tag at its C terminus (H-tag; Supplementary Fig. S1a ). Unlike the virus possessing the wild-type (wt) H protein, this virus did not form syncytia in Vero cells expressing the signalling lymphocyte activation molecule, a receptor for MV (Vero/hSLAM cells [10] ; Supplementary Fig. S1b ), presumably because the added tag adversely affected the interaction of the H protein with the receptor and/or the F protein. However, after a few passages the virus started to cause cell-to-cell fusion, and two independent three-time-passaged stocks (P3-1 and P3-2) produced large syncytia ( Fig. 1a ). Viruses were plaque-purified from these stocks, and their H, F and matrix (M) genes encoding the proteins involved in membrane fusion were subjected to sequence analysis after reverse transcription (RT)-PCR of RNA isolated from infected cells. In the F protein, the P3-1 virus stock had the N462K substitution, whereas the P3-2 stock had the G264R substitution. There was no amino-acid substitution in their H (H-tag) and M proteins. The F(N462K) protein has already been reported to exhibit enhanced fusion activity [11] . 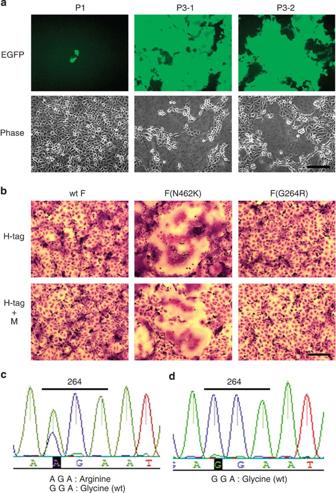Figure 1: Discrepancy between results from a recombinant virus and plasmid-mediated fusion assay. (a) Vero/hSLAM cells were infected with the P1 stock (passaged once) and two P3 stocks (P3-1 and P3-2) of the recombinant MV possessing the H-tag protein. At 2 days post-infection, the cells were observed under a fluorescence or phase-contrast microscope. (b) Vero/hSLAM cells were transfected with expression plasmids encoding H-tag and wt F or mutant F proteins, without (upper) or with (lower) that encoding the M protein. At 36 h post-transfection, cells were subjected to Giemsa staining and observed under a light microscope. (c,d) Sequence data of plaque-purified viruses from P3-2 (c) and P3-1 (d) stocks. Scale bars, 200 μm. Figure 1: Discrepancy between results from a recombinant virus and plasmid-mediated fusion assay. ( a ) Vero/hSLAM cells were infected with the P1 stock (passaged once) and two P3 stocks (P3-1 and P3-2) of the recombinant MV possessing the H-tag protein. At 2 days post-infection, the cells were observed under a fluorescence or phase-contrast microscope. ( b ) Vero/hSLAM cells were transfected with expression plasmids encoding H-tag and wt F or mutant F proteins, without (upper) or with (lower) that encoding the M protein. At 36 h post-transfection, cells were subjected to Giemsa staining and observed under a light microscope. ( c , d ) Sequence data of plaque-purified viruses from P3-2 ( c ) and P3-1 ( d ) stocks. Scale bars, 200 μm. Full size image We evaluated the role of these substitutions in the fusion activity of the viruses. Vero/hSLAM cells transfected with plasmids encoding H-tag and F(N462K) proteins, but not those with plasmids encoding H-tag and wt F proteins, formed extensive syncytia, as expected ( Fig. 1b ). However, no syncytia were detected in cells transfected with plasmids encoding H-tag and F(G264R) proteins. Co-expression of the M protein did not affect syncytium formation ( Fig. 1b ). Thus, there was a discrepancy between the phenotype of the P3-2 virus and the result of the plasmid-mediated fusion assay. We then rechecked the sequence data for the P3-2 virus, and found two overlapping peaks corresponding to amino-acid position 264 in the F gene of the P3-2 virus ( Fig. 1c ), but not in that of the P3-1 virus ( Fig. 1d ). The major peak indicated R264, whereas the minor one indicated the wt G264 (overlooked in our initial examination), suggesting that the P3-2 virus contained two types of genomes differing in the F gene. As paramyxoviruses are known to have the ability to include several genomes in one viral particle, called polyploidy [12] , [13] , [14] , our observation is not unexpected. A mixture of two F protein variants exhibits a new phenotype Next, we transfected Vero/hSLAM cells with plasmids encoding H-tag, wt F and F(G264R) proteins, and found syncytium formation in transfected cells ( Fig. 2a ). The result indicates that wt F and F(G264R) proteins together, but not individually, can mediate membrane fusion in conjunction with the H-tag protein. We then performed the fusion assay at different temperatures. At 30 °C, syncytia were observed in Vero/hSLAM cells expressing H-tag and F(G264R) proteins, but not in those expressing H-tag and wt F proteins ( Fig. 2b ). On the other hand, syncytia were formed in Vero/hSLAM cells expressing H-tag and wt F proteins after 10 min of incubation at 50 °C ( Fig. 2c ). It seems that temperature-dependent functions of wt F and F(G264R) proteins are neutralized by mixing them, as the combined F proteins functioned at 37 °C. 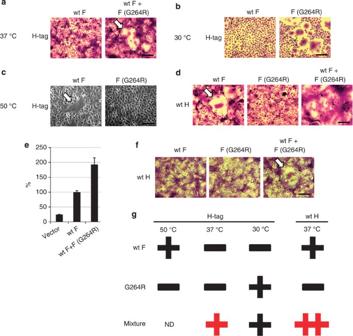Figure 2: A mixture of wt F and F(G264R) proteins exhibits a new phenotype. (a–c) Vero/hSLAM cells were transfected with expression plasmids encoding H-tag and wt F and/or F(G264R) proteins at 37 °C (a,c) or 30 °C (b). At 36 h post-transfection, the cells were subjected to Giemsa staining and observed under a light microscope (a,b) or, at 24 h post-transfection, cells were incubated at 50 °C for 10 min, and observed under a phase-contrast microscope (c). (d,f) Vero/hSLAM (d) and Vero (f) cells were transfected with expression plasmids encoding wt H and wt F and/or F (G264R) proteins at 37 °C. (e) Cell fusion levels with expression plasmids encoding H and F proteins were determined using the quantitative fusion assay. The activity obtained with the wt F protein was set to 100%. An empty vector was used as a negative control. Error bars, standard deviations. (g) Summary of the fusion activities of wt F protein, F(G264R) protein and their mixture. ND, not done. Scale bars, 200 μm (fora,b,d,f) or 100 μm (forc). White arrows indicate syncytia (a,c,d,f). Figure 2: A mixture of wt F and F(G264R) proteins exhibits a new phenotype. ( a – c ) Vero/hSLAM cells were transfected with expression plasmids encoding H-tag and wt F and/or F(G264R) proteins at 37 °C ( a , c ) or 30 °C ( b ). At 36 h post-transfection, the cells were subjected to Giemsa staining and observed under a light microscope ( a , b ) or, at 24 h post-transfection, cells were incubated at 50 °C for 10 min, and observed under a phase-contrast microscope ( c ). ( d , f ) Vero/hSLAM ( d ) and Vero ( f ) cells were transfected with expression plasmids encoding wt H and wt F and/or F (G264R) proteins at 37 °C. ( e ) Cell fusion levels with expression plasmids encoding H and F proteins were determined using the quantitative fusion assay. The activity obtained with the wt F protein was set to 100%. An empty vector was used as a negative control. Error bars, standard deviations. ( g ) Summary of the fusion activities of wt F protein, F(G264R) protein and their mixture. ND, not done. Scale bars, 200 μm (for a , b , d , f ) or 100 μm (for c ). White arrows indicate syncytia ( a , c , d , f ). Full size image The fusion assay was also performed by co-expressing the wt H protein in place of the H-tag protein ( Fig. 2d ). Syncytia were observed in Vero/hSLAM cells expressing wt H and wt F proteins, but not in those expressing wt H and F(G264R) proteins. However, Vero/hSLAM cells expressing wt H, wt F and F(G264R) proteins formed larger syncytia than those expressing wt H and wt F proteins, suggesting that the combined wt F and F(G264R) proteins exhibit enhanced fusion activity as compared with the wt F protein alone. Quantitative fusion assay confirmed this synergistic effect ( Fig. 2e ). Interestingly, when both wt F and F(G264R) proteins were present, even receptor-negative Vero cells developed syncytia ( Fig. 2f ; discussed below). Taken together, these results indicate that the mixed F proteins exhibit a new phenotype different from either wt F or F(G264R) protein ( Fig. 2g ). The F protein of paramyxoviruses, including MV, is known to form functional trimers [15] , [16] . Therefore, hetero-oligomeric proteins exhibiting a new phenotype may be formed when wt F and F(G264R) proteins are co-expressed. In fact, an co-immunoprecipitation assay revealed the complex formation between wt F and F(G264R) proteins ( Supplementary Fig. S2a ). Fusion assays were performed at various ratios of the plasmid encoding the wt F protein to that encoding the F(G264R) protein ( Supplementary Fig. S3 ). Several small syncytia were formed in Vero/hSLAM cells transfected with the 9:1 ratio of the plasmids, whereas syncytia were more extensively observed in those transfected with the 5:5 or 1:9 ratio. The results indicate that smaller amounts of the wt F protein compared with the F(G264R) protein were enough to induce efficient membrane fusion. It is thus likely that the heterotrimer with one wt F and two F(G264R) monomers has more fusogenicity than those with other combinations of monomers. On the basis of these data, we propose a possible model for the new phenotype of the combined F proteins ( Supplementary Fig. S4 ). The binding of the H protein to a cellular receptor triggers conformational changes of the F protein from the pre- to the post-fusion form during membrane fusion [9] . In our model, the conformational stability of its pre-fusion form has to be appropriate for the F protein to exhibit fusion activity upon receptor binding by the H protein. If the pre-fusion form of the F protein is too stable, receptor binding may not be able to trigger conformational changes in the F protein required for membrane fusion. This probably applies to the wt F protein acting in conjunction with the H-tag protein at 37 °C. On the other hand, if its stability is too low, as exemplified by the F(G264R) protein at 37 °C, the pre-fusion form may undergo an inappropriate folding before receptor binding, precluding the conformational changes required for membrane fusion. However, the wt F and F(G264R) proteins may induce membrane fusion in conjunction with the H-tag protein at 50 °C (due to reduced stability at a higher temperature) and 30 °C (due to increased stability at a lower temperature), respectively. Mixing the wt F and F(G264R) proteins may produce heterotrimers between these two types of F proteins, which presumably have the intermediate stability between wt F and F (G264R) proteins. We examined expression levels of the F proteins in transfected cells by western blot analysis ( Supplementary Fig. S2b ). The expression level of the wt F protein was reduced when it was co-expressed with the F(G264R) protein instead of expressed alone. Furthermore, the expression level of the F(G264R) protein as produced singly was increased at 30 °C compared with that at 37 °C. Although expression levels of the F protein may not completely reflect the conformational stability of the pre-fusion form of the protein, these results are consistent with the above model. Our model nicely explains why syncytium formation was observed at 37 °C, when both F proteins were expressed, but further studies are required to consolidate this model. Previously, Boulay et al. [17] reported that different influenza virus hemagglutinins formed mixed heterotrimers, which exhibited the intermediate property of the acid-induced activation. However, influenza virus usually does not have polyploidy, and these influenza virus hemagglutinin heterotrimers did not exhibit a new phenotype, unlike the MV F protein heterotrimes reported in the present study. Viruses carrying mixed genomes exhibit a new phenotype To validate our findings, we generated the recombinant MV containing these two types of genomes and examined its phonotype. One full-length genome plasmid carried the wt F gene and red fluorescent DsRed gene, and the other had the F(G264R) gene and EGFP gene ( Fig. 3a ). When both full-length genome plasmids were mixed and used to generate recombinant viruses (mixed genome viruses), infected cells formed syncytia expressing both DsRed and EGFP ( Fig. 3b ). The cells expressing either DsRed or EGFP (that is, cells infected with viruses containing only a single type of genome) did not form syncytia ( Supplementary Fig. S5 ). By contrast, when either full-length genome plasmid was used to generate recombinant viruses, syncytium formation was rarely, if any, observed ( Fig. 3b ). The recombinant virus recovered from syncytia was used to infect cells, and its F gene was sequenced after RT-PCR of RNA isolated from the cells. It retained two different sequences at position 264 of the F protein ( Fig. 3c ), indicating that the syncytium-forming phenotype of the P3-2 virus is indeed dependent on a mixture of the two types of genomes. Furthermore, a linear relationship was found between the numbers of plaques and dilution rates, by the plaque assay of the same stock of the mixed genome virus ( Supplementary Fig. S6 ). This result indicates that most individual MV particles of the mixed genome virus contain both types of genomes. 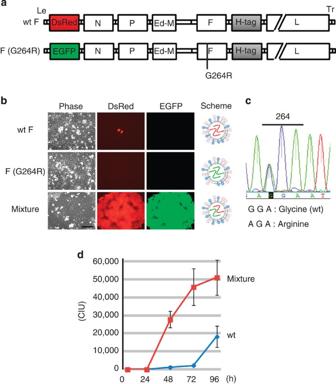Figure 3: Viruses carrying the two different genomes exhibit a new phenotype. (a) Full-length genome plasmids used for recovery of recombinant viruses. Le, leader. N, nucleocapsid. P, phospho. Ed-M, Edmonston M. L, large. Tr, trailer. (b) Cells infected with recombinant viruses prepared with the full-length genome plasmid carrying the wt F gene, one carrying the mutant F(G264R) gene or both (mixture). The genomes of respective recombinant viruses are schematically shown. Cells were observed under a phase-contrast and a fluorescence microscope. (c) A virus was isolated from syncytium obtained with the mixture of the full-length genome plasmids, and its F gene sequence was determined. (d) Vero/hSLAM cells were infected with the virus carrying the wt F protein alone (wt) or the mixed genome virus (mixture) at a multiplicity of infection of 0.001. The cells and supernatant were collected 4, 24, 48, 72 and 96 h post-infection, and the titres of collected samples (expressed as cell infectious unit (CIU)) were determined in Vero/hSLAM cells. Error bars, standard deviations. Scale bars, 200 μm. Figure 3: Viruses carrying the two different genomes exhibit a new phenotype. ( a ) Full-length genome plasmids used for recovery of recombinant viruses. Le, leader. N, nucleocapsid. P, phospho. Ed-M, Edmonston M. L, large. Tr, trailer. ( b ) Cells infected with recombinant viruses prepared with the full-length genome plasmid carrying the wt F gene, one carrying the mutant F(G264R) gene or both (mixture). The genomes of respective recombinant viruses are schematically shown. Cells were observed under a phase-contrast and a fluorescence microscope. ( c ) A virus was isolated from syncytium obtained with the mixture of the full-length genome plasmids, and its F gene sequence was determined. ( d ) Vero/hSLAM cells were infected with the virus carrying the wt F protein alone (wt) or the mixed genome virus (mixture) at a multiplicity of infection of 0.001. The cells and supernatant were collected 4, 24, 48, 72 and 96 h post-infection, and the titres of collected samples (expressed as cell infectious unit (CIU)) were determined in Vero/hSLAM cells. Error bars, standard deviations. Scale bars, 200 μm. Full size image Next, we compared the growth of the virus containing the wt F gene with that of the mixed genome virus in Vero/hSLAM cells. As expected, the mixed genome virus grew faster than the virus containing the wt F gene alone ( Fig. 3d ). This growth advantage must have allowed the evolution of the recombinant MV with the H-tag protein, producing the mixed genome virus in Vero/hSLAM cells. We also examined viral spread in hamster brains, which do not have efficient receptors for MV. For this experiment, we newly recovered recombinant MVs expressing the wt H protein, not the H-tag protein, and 7-day-old hamsters were inoculated intracerebrally with the virus containing the wt F gene or the mixed genome virus ( Fig. 4a ). Six days after inoculation, hamster brains were collected, and examined under fluorescence and stereoscopic microscopes ( Fig. 4b ). The mixed genome virus spread in the brains (probably by cell-to-cell fusion), while the virus containing the wt F gene alone infected individual cells, but did not produce syncytia. Viruses recovered from the brain inoculated with the mixed genome virus still had both types of genomes ( Supplementary Fig. S7 ). Thus, ‘cooperation’ of two different genomes can provide a virus with the ability to propagate in non-host, receptor-negative tissues, in which the wt virus does not propagate. 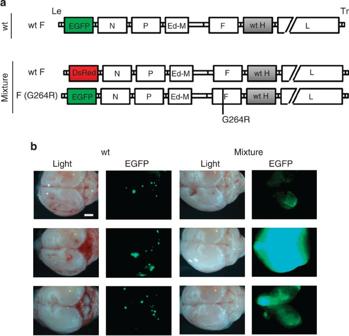Figure 4: Efficient spread of the mixed genome virus in hamster brains. (a) Full-length genome plasmids used for recovery of recombinant viruses expressing the wt H protein. (b) Seven-day-old hamsters were inoculated intracerebrally with the virus carrying the wt F protein alone (wt) or the mixed genome virus (mixture). Six days after inoculation, their brains were collected and observed under stereoscopic and fluorescence microscopes. Scale bars, 2 mm. Figure 4: Efficient spread of the mixed genome virus in hamster brains. ( a ) Full-length genome plasmids used for recovery of recombinant viruses expressing the wt H protein. ( b ) Seven-day-old hamsters were inoculated intracerebrally with the virus carrying the wt F protein alone (wt) or the mixed genome virus (mixture). Six days after inoculation, their brains were collected and observed under stereoscopic and fluorescence microscopes. Scale bars, 2 mm. Full size image In the present study, a mutant cooperatively acting with the wt was observed. This mutant F(G264R) protein enhances membrane fusion and viral growth only when expressed together with the wt F protein. Therefore, the viral genetic composition changes from a single type of genome to a mixture of two different genomes. It should be noted that this phenomenon is different from complementation, because the two genomes do not complement each other, but produce a new phenotype through ‘cooperation’. Is ‘cooperation’a common event? We have passaged the recombinant MV expressing the H-tag protein in Vero/hSLAM cells, and recovered, altogether, eight viruses that regained the ability to induce membrane fusion, including P3-1 and P3-2 described in this study. Among them, six viruses had the single substitutions that endowed their F proteins with increased fusion activity, such as F(N462K). One virus had the genome encoding the F protein with the N92D and G264R substitutions, as well as that encoding the wt F protein, such as the P3-2 stock. This virus was also found to cause syncytia through ‘cooperation’ of the two genomes. Thus, ‘cooperation’ may not be common, but not very rare, either (two out of eight events in this example). Furthermore, the mixed genome virus expressing wt F and F(G264R) proteins retained its genomic composition even after five passages (data not shown), suggesting that ‘cooperation’ is a stable phenomenon, at least in this case. Does ‘cooperation’ occur in the natural world? Long-term transmission of defective RNA genomes has been reported in dengue virus isolates, although the mechanism remains to be elucidated [18] . ‘Cooperation’ may be an explanation for this phenomenon. Furthermore, cooperation could occur for any proteins forming functional oligomers. We suspect that protein complexes containing heterogeneous subunits necessary for their function might have arisen through the cooperation between wt and variant alleles. Further studies on many viruses, especially paramyxoviruses in which polyploidy occurs, may reveal more examples of cooperation. MV can infect various cultured cells independent of known receptors albeit at low efficiencies (100- to 1000-fold lower than that of SLAM-dependent infection) [19] . This inefficient infection has been postulated to account for MV infection of neurons in human patients [20] . This mode of infection presumably occurs because the F protein may sometimes be activated when the H protein interacts with molecules other than known receptors. Enhanced fusion activity of the F protein, as exhibited by the adapted MV in the present study, may increase the rate of this activation, and allow MV to infect receptor-negative cells, such as Vero cells ( Fig. 2f ), hamster brain cells ( Fig. 4b ) and neurons in patients with subacute sclerosing panencephalitis. Furthermore, virus populations with mixed genomes could be evolutionary intermediates, which with time may adapt to infection in receptor-negative cells of host or non-host species. Viruses Recombinant viruses based on the IC-B strain [19] were recovered as described previously [21] . The M gene was replaced by the Edmonston strain M gene to facilitate virus particle formation [22] . Full-length genome plasmids p(+)HHRz-MV323-DsRed(H-tag/wtF) and p(+)HHRz-MV323-EGFP(H-tag/F(G264R)) were mixed when recovering the recombinant virus containing two types of genomes. Fusion assay Cells were transfected with expression plasmids encoding MV H and F proteins, together with or without that encoding the Edmonston M protein. For the quantitative fusion assay, HEK293T cells were co-transfected with expression plasmids encoding MV H, MV F, firefly-luciferase and Renilla -luciferase. At 5-h post-transfection, the cells were mixed with Vero/hSLAM cells expressing the T7 RNA polymerase (Vero/hSLAM-T7). The Renilla -luciferase gene is encoded downstream of the T7-promoter, and its transcription is activated by fusion between Vero/hSLAM-T7 and HEK293T cells. At 24 h post-transfection, activities of both luciferases in the cells were analysed using Dual-luciferase reporter assay system (Promega), according to the manufacturer’s instructions. Renilla -luciferase activity was divided by firefly-luciferase activity (directed by the herpes simplex virus thymidine kinase promoter) to correct transfection efficiency. Immunoprecipitation and western blot analysis HEK293T cells were co-transfected with expression plasmids encoding the HA-tagged wt F protein (wt F-HA) and/or FLAG-tagged F(G264R) protein (F(G264R)-FLAG). The cells were lysed in a radioimmunoprecipitation assay buffer (1% NP-40, 150 mM NaCl, 10 mM Tris–HCl, pH 7.4, 1% sodium deoxycholate, 0.1% SDS), followed by centrifugation. The supernatants were pre-cleared by protein A-Sepharose (GE Healthcare AB), and a small amount of each supernatant was collected as a cell-lysate sample. The rest of the supernatant was incubated with anti-FLAG M2 monoclonal antibody (Sigma-aldrich)-treated protein A-Sepharose. The immunoprecipitates were collected by centrifugation and washed three times with radioimmunoprecipitation assay buffer. The supernatants were also collected for determining protein expression levels ( Supplementary Fig. S2b ). The samples were analysed by SDS–polyacrylamide gel electrophoresis and immunoblotted with an anti-HA-tag antibody or anti-FLAG antibody. How to cite this article: Shirogane, Y. et al. Cooperation between different RNA virus genomes produces a new phenotype. Nat. Commun. 3:1235 doi: 10.1038/ncomms2252 (2012).